Selection on haemagglutinin imposes a bottleneck during mammalian transmission of reassortant H5N1 influenza viruses The emergence of human-transmissible H5N1 avian influenza viruses poses a major pandemic threat. H5N1 viruses are thought to be highly genetically diverse both among and within hosts; however, the effects of this diversity on viral replication and transmission are poorly understood. Here we use deep sequencing to investigate the impact of within-host viral variation on adaptation and transmission of H5N1 viruses in ferrets. We show that, although within-host genetic diversity in haemagglutinin (HA) increases during replication in inoculated ferrets, HA diversity is dramatically reduced upon respiratory droplet transmission, in which infection is established by only 1–2 distinct HA segments from a diverse source virus population in transmitting animals. Moreover, minor HA variants present in as little as 5.9% of viruses within the source animal become dominant in ferrets infected via respiratory droplets. These findings demonstrate that selective pressures acting during influenza virus transmission among mammals impose a significant bottleneck. Avian H5N1 influenza viruses sporadically infect humans with a lethality rate approaching 60% among confirmed cases; however, they have not yet acquired the capacity for sustained human-to-human transmission [1] . Recent work has demonstrated that a limited number of mutations can enable droplet transmission of H5N1 influenza viruses among mammals, heightening concern that a future pandemic could arise from the acquisition of a transmissible phenotype by H5N1 viruses currently circulating in nature [2] , [3] . The dynamics governing the emergence of pandemic influenza viruses are not completely defined. Historically, most influenza pandemics have been caused by viruses with HAs against which the human population had limited pre-existing immunity [4] , [5] , [6] , [7] . The spread of H5N1 viruses in wild birds and poultry on several continents and human H5N1 infections have focused attention on H5N1 viruses as potential sources of future pandemics. Despite widespread circulation of H5N1 viruses and significant human contact with infected poultry and birds, the number of documented human cases of H5N1 infection is relatively low, and human-to-human transmission of H5N1 viruses is rare [8] , [9] . The likelihood of an H5N1 pandemic in humans is largely determined by factors affecting the emergence of viruses that efficiently replicate in humans and transmit person-to-person [10] , [11] , [12] , [13] , [14] , [15] , [16] . Influenza viruses exist in the host as a diverse collection of genetically linked variants that arise because of the combined effects of error-prone genome replication, rapid replication kinetics and large population sizes [17] , [18] . The within-host viral population structure reflects a balance between the generation of diversity through mutation and its loss through selection. The resulting ‘swarm’ of genetic variants can rapidly adapt in response to selective pressures. The rate at which influenza genetic diversity is generated within hosts and the degree to which it is maintained upon transmission are therefore two main parameters determining the likelihood with which mammalian-transmissible viruses might emerge in nature. We recently examined the molecular features that enable mammalian transmission of H5N1 influenza viruses. HA has a major role in restricting influenza virus host range, in part because of receptor specificity [19] . HA proteins of avian H5N1 viruses preferentially recognize sialic acid linked to galactose by α2,3-linkages (Siaα2,3 Gal), whereas human influenza isolates preferentially recognize α2,6-linked sialic acid (Siaα2,6 Gal) [20] . In previous work [2] , we identified two amino-acid substitutions (N224K and Q226L) that cooperatively enabled Siaα2,6 Gal human-type receptor binding by an HA protein derived from the pathogenic avian virus A/Vietnam/1203/2004 (VN1203; H5N1). We created reassortant viruses bearing VN1203 HA genes encoding N224K and Q226L substitutions, with the seven remaining segments derived from A/California/04/2009 (CA04; H1N1), and evaluated their replication in ferrets. An additional substitution at HA amino-acid position 158 (N→D) was associated with increased virus titres in ferret nasal turbinates. To evaluate transmissibility in ferrets, we therefore first used a virus isolate bearing all three mutations in HA (N158D/N224K/Q226L; herein called VN1203-HA(3)-CA04). In these experiments, ‘index’ ferrets were inoculated intranasally with 10 6 plaque-forming units (p.f.u.) of virus stock. One day later, each infected ferret was paired with an uninfected ‘contact’ ferret placed in an adjacent cage that prevented direct contact between the animals but permitted airborne droplet transmission of the influenza virus. VN1203-HA(3)-CA04 was transmitted between animals in two of six ferret pairs. During replication of this virus in a contact animal, an additional T318I amino-acid substitution was detected. The N158D/N224K/Q226L/T318I virus (herein called VN1203-HA(4)-CA04) had an improved transmission efficiency, being transmitted between animals in four of the six ferret pairs [2] . Here we evaluate the impact of within-host viral genetic diversity on the replication and transmission of H5N1 reassortant viruses described in our previous study [2] . Using deep sequencing, we assess viral genetic variation during the infection of inoculated ferrets and in contact ferrets infected via respiratory droplet transmission. We report that HA segment diversity increases rapidly following intranasal inoculation of ferrets, resulting in a genetically diverse population of viruses in each infected host. In contrast, we show that there is a transmission-associated bottleneck in which only a limited subset of the HA segments is transmitted to contact ferrets. Furthermore, we find that even variants present at frequencies of as little as 5.9% in one infected animal can be transmitted via respiratory droplets. This report establishes that selective forces acting on the HA segment impose a significant bottleneck during respiratory droplet transmission of reassortant H5 influenza viruses. Low sequence diversity in transmissible H5N1 virus stocks Here we use deep sequencing to investigate H5N1 influenza virus variation during replication and transmission in mammals, using archived RNA samples that were collected from ferrets during the previous study [2] (see Supplementary Fig. S1 for ferret experiment outline). Note that no new virus transmission experiments were conducted for this study. We emphasize that these studies use avian–human reassortant viruses that encode an avian H5 HA protein in the background of a human H1N1 virus isolate that is likely already well-adapted to growth and transmission in mammals. Whereas the HA protein has a central role in the adaptation of avian influenza viruses to mammalian hosts, proteins encoded by other gene segments can also influence avian influenza virus adaptation and replication in mammals [11] , [13] , [16] , [21] , [22] . Studies using fully avian viruses may therefore yield results that differ from those described here. We use the Illumina MiSeq instrument in these experiments because of its high throughput and low error rate [23] . Data generated by this instrument are largely free of the homopolymer-associated indel errors, which are common to other sequencing platforms [24] . We first characterized the nucleotide sequence diversity in the HA gene of VN1203-HA(3)-CA04 and VN1203-HA(4)-CA04 virus stocks, which were collected after a single passage in Madin–Darby canine kidney (MDCK) cells ( Fig. 1 ). As expected, the mutations previously reported in association with the transmissible phenotype of these H5N1 viruses are present at or near 100% fixation ( Fig. 1 ). The majority of HA nucleotide diversity in both viruses is present at <1% per site (that is, for a given nucleotide position, fewer than 1% of sequence ‘reads’ varied from the consensus residue). However, multiple nonsynonymous single nucleotide polymorphisms (SNPs) are present at frequencies between 1 and 99% in both stock viruses. VN1203-HA(3)-CA04 stock virus SNPs are located at nucleotide 53 (1.5%, encoding an alanine-to-threonine substitution), 215 (1.1%, encoding a valine-to-leucine substitution), 788 (3.2%, encoding an alanine-to-serine substitution) and 1,020 (1.9%, encoding a threonine-to-isoleucine substitution). VN1203-HA(4)-CA04 stock virus SNPs are located at nucleotide 788 (4.4%, encoding an alanine-to-threonine amino-acid substitution) and 1,580 (6.6%, encoding a glutamate-to-lysine amino-acid substitution). We also note a synonymous substitution at HA nucleotide 1,018 in VN1203-HA(3)-CA04 (4.1%). Deep sequencing of NA and M segments from both stock viruses reveals few SNPs above 1% frequency ( Supplementary Fig. S2A,B ). 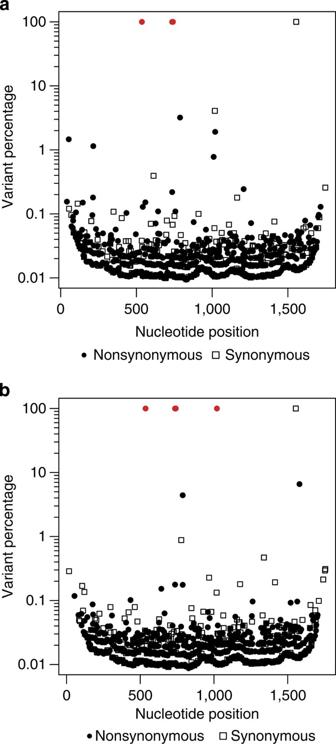Figure 1: Deep sequencing reveals low sequence variation in haemagglutinin of influenza virus stocks. We used deep sequencing to probe the nucleotide diversity of the (a) VN1203-HA(3)-CA04 and (b) VN1203-HA(4)-CA04 virus stocks used in mammalian transmission experiments. Individual HA sequence reads were mapped to a consensus HA sequence derived from the isolate A/Vietnam/1203/2004 (H5N1). SNPs were enumerated as described in Methods. No variants were detected below 0.01%. The frequency of variants at each site is presented as either closed circles (nonsynonymous substitutions) or open squares (synonymous substitutions). Mutations previously reported in association with mammalian transmission are highlighted in red: VN1203-HA(3)-CA04: N158D (nt 536), N224K (nt 736) and Q226L (nt 741) and VN1203-HA(4)-CA04: N158D (nt 536), N224K (nt 736), Q226L (nt 741) and T318I (nt 1,020). A synonymous mutation at nucleotide position 1555 that was not present in the plasmid used to generate viruses by reverse genetics was detected in each virus stock after harvest and before infection of ferrets. Figure 1: Deep sequencing reveals low sequence variation in haemagglutinin of influenza virus stocks. We used deep sequencing to probe the nucleotide diversity of the ( a ) VN1203-HA(3)-CA04 and ( b ) VN1203-HA(4)-CA04 virus stocks used in mammalian transmission experiments. Individual HA sequence reads were mapped to a consensus HA sequence derived from the isolate A/Vietnam/1203/2004 (H5N1). SNPs were enumerated as described in Methods. No variants were detected below 0.01%. The frequency of variants at each site is presented as either closed circles (nonsynonymous substitutions) or open squares (synonymous substitutions). Mutations previously reported in association with mammalian transmission are highlighted in red: VN1203-HA(3)-CA04: N158D (nt 536), N224K (nt 736) and Q226L (nt 741) and VN1203-HA(4)-CA04: N158D (nt 536), N224K (nt 736), Q226L (nt 741) and T318I (nt 1,020). A synonymous mutation at nucleotide position 1555 that was not present in the plasmid used to generate viruses by reverse genetics was detected in each virus stock after harvest and before infection of ferrets. Full size image HA sequence variation increases with time in index animals The presence of detectable low-level sequence diversity in HA, NA and M prompts us to consider the potential impact of within-host viral variation on adaptive processes in ferrets. To follow changes in the viral population in inoculated ferrets and after transmission to naive contact ferrets, we analyse viruses isolated from nasal wash samples collected from only the ferret pairs in which H5N1 reassortant viruses were transmitted between animals in our previous experiments [2] . To test for evidence of selective pressures favouring viruses bearing specific mutations in the avian HA segment, we evaluate all individual SNPs occurring at a frequency of ≥1% in stock virus preparations or in any single sample from one or more of the infected index ferrets ( Fig. 2 ). To confirm that SNPs detectable above this threshold were not the result of sequencing or PCR errors, we deep-sequenced plasmid DNA and an in vitro transcription product encoding a fragment of the influenza virus M gene (see Methods for details). In these samples, nucleotide variation did not exceed 0.4% at any position, suggesting that our threshold of ≥1% ensures that only bona fide SNPs are considered in our analyses ( Supplementary Fig. S2C,D ). 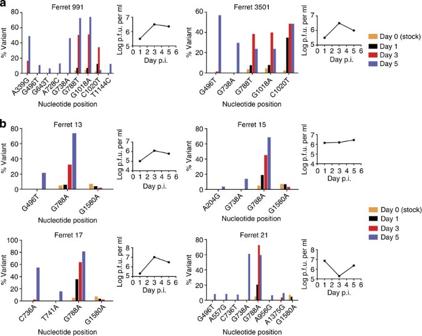Figure 2: Within-host selection of HA segments harbouring specific single nucleotide polymorphisms. Viral RNA recovered in nasal wash samples collected from ferrets at different time points following intranasal infection with the indicated viruses was used to measure HA segment variation by deep sequencing. Bar graphs depict changing frequencies of specific SNPs during the infection of index ferrets with (a) VN1203-HA(3)-CA04 or (b) VN1203-HA(4)-CA04 viruses. Number of sequences used to calculate SNP frequencies ranged fromn=198–15,206 for VN1203-HA(3)-CA04 andn=111 to 11,411 for VN1203-HA(4)-CA04. This analysis focused on SNPs detected in at least 1% of virus sequences in stock viruses or in one or more samples collected from any ferret at any time point. Each SNP was nonsynonymous, with the exception of a synonymous SNP at nucleotide position 1018. Inset line graphs depict virus titres in nasal wash samples collected from each index ferret at the indicated time point. Virus titres were measured using a standard plaque assay on MDCK cells. Figure 2: Within-host selection of HA segments harbouring specific single nucleotide polymorphisms. Viral RNA recovered in nasal wash samples collected from ferrets at different time points following intranasal infection with the indicated viruses was used to measure HA segment variation by deep sequencing. Bar graphs depict changing frequencies of specific SNPs during the infection of index ferrets with ( a ) VN1203-HA(3)-CA04 or ( b ) VN1203-HA(4)-CA04 viruses. Number of sequences used to calculate SNP frequencies ranged from n =198–15,206 for VN1203-HA(3)-CA04 and n= 111 to 11,411 for VN1203-HA(4)-CA04. This analysis focused on SNPs detected in at least 1% of virus sequences in stock viruses or in one or more samples collected from any ferret at any time point. Each SNP was nonsynonymous, with the exception of a synonymous SNP at nucleotide position 1018. Inset line graphs depict virus titres in nasal wash samples collected from each index ferret at the indicated time point. Virus titres were measured using a standard plaque assay on MDCK cells. Full size image During infection of ferrets, viruses encoding mutations away from the reference sequence at nucleotide 788, a site at which we observed low-frequency SNPs in both stock viruses, reach 30% frequency or greater in each of the six index ferrets examined. A G→T SNP at nucleotide 788 encoding an alanine-to-serine amino-acid substitution is present in the two ferrets infected with VN1203-HA(3)-CA04, and a G→A SNP at nucleotide 788 encoding an alanine-to-threonine substitution is present in the four ferrets infected with VN1203-HA(4)-CA04 ( Fig. 2 ). The respective SNPs are present in the VN1203-HA(3)-CA04 stock virus at 3.2% and in the VN1203-HA(4)-CA04 stock virus at 4.4% ( Table 1 ). Nucleotide 788 is the first position of codon 238 of the mature H5 HA protein (amino acid 242 by H3 numbering) and is located within the molecule’s globular head. Each of these mutations creates a potential signal for glycosylation of the upstream asparagine residue at amino-acid position 236 (240 by H3 numbering). The frequency of variant nucleotides at position 788 in index animals is positively correlated with day post infection ( r =0.857; P<0.001, Pearson’s correlation coefficient), showing a significant increase in the variant nucleotide over time ( Supplementary Fig. S3 ). These results indicate that amino-acid substitutions away from the consensus alanine at HA position 238 are strongly favoured during the replication of H5N1 reassortant viruses in index ferrets that transmitted viruses to their contacts. Although viruses with both wild-type and variant sequences at nucleotide 788 are clearly replication-competent in vivo , our data do not allow us to draw further conclusions about the action of selection on this position in contact animals. Future work will be needed to fully characterize the effects of amino-acid substitutions at HA position 238 on the replication fitness of H5N1 viruses in mammals. Table 1 Single nucleotide polymorphisms detected in HA segments of viral populations recovered from infected ferrets. Full size table A number of additional SNPs change markedly in frequency during the infection of index ferrets with either virus ( Fig. 2 ). In some cases, SNPs that change in frequency during infection of ferrets are detectable at frequencies between 1 and 5% in viral stocks (for example, SNPs at nucleotide 788 of VN1203-HA(3)-CA04 and VN1203-HA(4)-CA04 virus stocks in Fig. 2a,b ). Multiple SNPs in both viruses rapidly increase to frequencies above 20% in index animals (for example, SNPs at nucleotides 738, 788 and 1020 in virus VN1203-HA(3)-CA04, Fig. 2a and at positions 736 and 788 in VN1203-HA(4)-CA04, Fig. 2b ), although variant SNPs decline in frequency in some index animals at very late time points. Overall, the reproducible increase in frequencies of nonsynonymous SNPs at sites such as nucleotide 788 in multiple index animals suggests that selection favours variant amino acids at these positions during virus replication in vivo. In contrast, the SNP located at nucleotide position 1580 in the VN1203-HA(4)-CA04 stock virus decreases in frequency following infection of each of the four index ferrets ( Fig. 2b ; ferrets 13, 15, 17 and 21), indicating that selection does not favour sequence variants at this position in vivo . Droplet transmission of a small number of HA variants To determine whether selective pressures might be acting during respiratory droplet transmission of H5N1 reassortant influenza viruses, we first compared the frequencies of HA SNPs in viruses replicating in index and contact ferrets. As shown in Fig. 2 , multiple HA SNPs arise and achieve frequencies up to 80% during infection of index ferrets with either virus. If infection of the contact results from the transfer of a representative sample of virus from the transmitting animal, one would expect to see similar HA SNP frequencies in the contact animal upon establishment of infection. Strikingly, however, HA sequences of the viral population replicating at the earliest detectable time point in contact animals do not reflect the frequencies of SNPs present in the paired index ferret near the time of transmission ( Fig. 3 and Supplementary Fig. S4 ; see Supplementary Fig. S1B for information on approximate timing of transmission). Instead, SNPs are either present at nearly 100% or almost completely absent following transmission, suggesting that the infection of contact animals is established by a virus population with a relatively homogeneous HA sequence. Indeed, even SNPs present as minor variants in index animals are found dominating the population replicating shortly after transmission in contact animals. For example, a lysine-to-asparagine substitution encoded by a SNP at nucleotide 643 (amino acid 193 by H3 numbering) is detected in 5.9% of viruses in the pair 1 index animal shortly before transmission, and this same substitution is present in virtually 100% of virus sequences detected shortly after transmission in the paired contact animal ( Fig. 3 , pair 1). 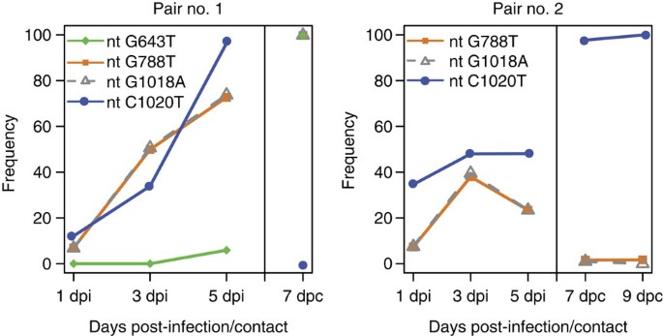Figure 3: Detection of HA SNPs early after infection in contact animals. HA gene segments accumulated diversity over time during replication in index animals, as demonstrated by the increasing frequency of substitutions at positions 643, 788, 1,018 and 1,020 in index animals infected with VN1203-HA(3)-CA04 (left-hand portion of each panel). Following transmission, the founding virus population in contact animals displayed a shift in SNP frequencies, such that SNPs were either nearly fixed in, or were absent from, the replicating virus population. A SNP detected in 5.9% of viruses in the pair 1 index animal shortly before transmission was present in nearly 100% of virus sequences shortly after transmission in the paired contact animal. Number of sequences used to calculate SNP frequencies ranged fromn=1,472 to 13,324. Figure 3: Detection of HA SNPs early after infection in contact animals. HA gene segments accumulated diversity over time during replication in index animals, as demonstrated by the increasing frequency of substitutions at positions 643, 788, 1,018 and 1,020 in index animals infected with VN1203-HA(3)-CA04 (left-hand portion of each panel). Following transmission, the founding virus population in contact animals displayed a shift in SNP frequencies, such that SNPs were either nearly fixed in, or were absent from, the replicating virus population. A SNP detected in 5.9% of viruses in the pair 1 index animal shortly before transmission was present in nearly 100% of virus sequences shortly after transmission in the paired contact animal. Number of sequences used to calculate SNP frequencies ranged from n= 1,472 to 13,324. Full size image The difference in HA sequence composition in contact ferrets compared with index ferrets following respiratory droplet-mediated transmission suggests that there is a severe bottleneck associated with transmission of these H5N1 viruses. To more closely evaluate the genetic composition of HA segments in the mixed viral populations in index and contact animals, we identified linkage relationships among SNPs detected during infection and after transmission. In this analysis, we take advantage of the fact that information about the physical linkage among SNPs of interest is preserved in a subset of sequence reads for each HA gene segment. This is possible because, in preparation for deep sequencing, amplified HA segments are randomly sheared into fragments with an average length of 500 nucleotides, which are sequenced from both ends. Therefore, the linkage of SNPs located in a defined window of ~500 nucleotides of the HA segment can be assessed in a subset of high-quality sequencing reads that covers the region of interest. Using this approach, we define the identity and frequency of various SNP combinations in HA segments present at each time point in the index and contact animals. We term each distinct combination of SNPs an HA ‘haplotype’. We confirmed the validity of this approach by cloning and sequencing a panel of full-length HA segments from representative samples ( Supplementary Table S1 ). In general, the number of HA haplotypes present in index animals increases throughout infection ( Fig. 4 ). By day 5 post infection, no single HA haplotype accounts for >50% of the HA segments detected in the viral population of any index animal, irrespective of the infecting virus stock, indicating that the HA genes of both viruses rapidly diversify in vivo ( Fig. 4 ). Whereas many of the identified HA haplotypes are detected in all index animals infected with either virus, some haplotypes are unique to particular animals, suggesting that stochastic processes, host genetics and/or other factors might have an impact on the within-host viral evolution. Collectively, these data demonstrate that the assemblage and frequency of HA haplotypes are dynamic during the infection of index animals with these H5N1 viruses, with a trend towards increasing HA haplotype diversity. 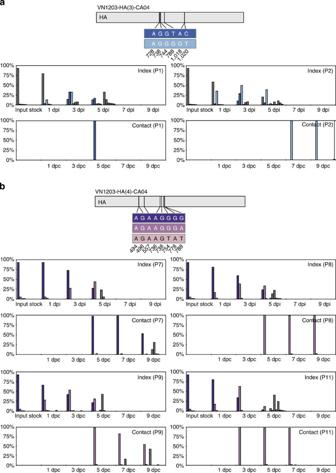Figure 4: Enumeration of HA segment haplotypes. To identify patterns of physically linked SNPs, we took advantage of the fact that paired-end deep sequencing provides ‘mate-paired’ reads that are separated by intervening sequences of varying length, allowing us to identify reads containing sites of interest that are linked on the same viral RNA. By analysing these reads, we identified linkage relationships among targeted SNPs and use the term ‘haplotype’ to denote a single unique combination of SNPs. SNPs used to define HA haplotypes are shown schematically above each panel. This analysis targeted nucleotides 728, 738, 744, 788, 1,018 and 1,020 in virus VN1203-HA(3)-CA04 (a) and nucleotides 494, 496, 557, 736, 754, 778 and 788 in virus VN1203-HA(4)-CA04 (b). We considered only haplotypes detected at or above a frequency of 1% of the total virus population. Transmission pairs are indicated as paired boxes, each with an index animal (above) and a contact animal (below). Thexaxis represents the sample collection time points for index or contact animals. Grey bars denote the frequencies of non-transmitting haplotypes. The frequencies of HA haplotypes implicated in transmission are coloured with the specific constellation of SNPs indicated in the schematic above each panel. Note that the minor haplotype detected at the first time point in which virus was recovered from the contact ferret of pairs 7 and 9 was also found in the paired index ferret. Number of sequences used to calculate haplotype frequencies ranged fromn=1,418 to 3,128 for VN1203-HA(3)-CA04 andn=540 to 1,050 for VN1203-HA(4)-CA04. Further details can be found inSupplementary Tables S2 and S3. Figure 4: Enumeration of HA segment haplotypes. To identify patterns of physically linked SNPs, we took advantage of the fact that paired-end deep sequencing provides ‘mate-paired’ reads that are separated by intervening sequences of varying length, allowing us to identify reads containing sites of interest that are linked on the same viral RNA. By analysing these reads, we identified linkage relationships among targeted SNPs and use the term ‘haplotype’ to denote a single unique combination of SNPs. SNPs used to define HA haplotypes are shown schematically above each panel. This analysis targeted nucleotides 728, 738, 744, 788, 1,018 and 1,020 in virus VN1203-HA(3)-CA04 ( a ) and nucleotides 494, 496, 557, 736, 754, 778 and 788 in virus VN1203-HA(4)-CA04 ( b ). We considered only haplotypes detected at or above a frequency of 1% of the total virus population. Transmission pairs are indicated as paired boxes, each with an index animal (above) and a contact animal (below). The x axis represents the sample collection time points for index or contact animals. Grey bars denote the frequencies of non-transmitting haplotypes. The frequencies of HA haplotypes implicated in transmission are coloured with the specific constellation of SNPs indicated in the schematic above each panel. Note that the minor haplotype detected at the first time point in which virus was recovered from the contact ferret of pairs 7 and 9 was also found in the paired index ferret. Number of sequences used to calculate haplotype frequencies ranged from n =1,418 to 3,128 for VN1203-HA(3)-CA04 and n =540 to 1,050 for VN1203-HA(4)-CA04. Further details can be found in Supplementary Tables S2 and S3 . Full size image The diversity of HA haplotypes in index ferrets is not reflected in the virus population found in contact animals following transmission ( Fig. 4 , Supplementary Tables S2 and S3 ). Instead, a single predominant HA haplotype is detected in each of the six contact ferrets at the earliest time point at which we recovered virus ( Fig. 4 , Supplementary Fig. S1B ). In VN1203-HA(3)-CA04-infected contacts, infection is established by a relatively monomorphic population of viruses possessing a single HA haplotype, although the specific transmitting HA haplotype differs between the two ferret pairs ( Fig. 4a ). Similar patterns are found in ferret pairs infected with VN1203-HA(4)-CA04. In contrast to the heterogeneous mixture of HA haplotypes present in index ferrets, the first samples of virus collected from contact animals contain either a single detectable HA haplotype ( Fig. 4b , pair 8 and pair 11), or a single predominant HA haplotype with a second detectable haplotype present at a low frequency ( Fig. 4b , pair 7 and pair 9, day 5). It is unclear whether the minority HA haplotypes detected early in contact ferrets are transmitted from the animals’ paired index ferrets or are derived from the more prevalent HA haplotype following the establishment of infection. Using the same approach, we also identify NA and M1 gene haplotypes during infection and after transmission (see Supplementary Tables S4 and S5 for NA and Supplementary Tables S6 and S7 for M1). Although multiple NA and M1 haplotypes are defined, the virus population in index ferrets is dominated by a single NA and M1 haplotype in each animal, with 2–5 minor variant haplotypes present at 1–5% ( Supplementary Tables S4 and S6 , respectively). In contrast to our observations for the HA segment, there is no narrowing of NA or M1 haplotype diversity after transmission. Together, these data show that there is a severe bottleneck in HA segment diversity associated with the transmission of H5N1 influenza viruses via respiratory droplets. As a result, infection is established in the contact host by a population of viruses with a single predominant HA haplotype that resembles only one of multiple haplotypes generated during viral replication in the infected transmitting animal. Transmission bottleneck is associated with selection on HA At least two non-mutually exclusive processes could cause a severe bottleneck during transmission. First, a low infectious dose could account for the diminution in HA sequence diversity during transmission if only one or a few viral particles establish infection in the new host, a situation commonly referred to as the founder effect. In this situation, natural selection would not act to favour the transmission of particular viruses, and we would expect to observe low genetic diversity in all viral gene segments immediately after transmission. Second, strong selective pressures could favour the transmission of viruses possessing particular HA haplotypes that confer improved transmission efficiency. In this situation, termed a ‘selective sweep’, diversity is reduced as natural selection eliminates viruses that are poorly adapted for transmission [25] . In a selective sweep acting on HA, we would therefore expect transmitted viruses to show a greater reduction in HA genetic diversity as compared with diversity in other gene segments. To determine the relative impact of these two processes, we measure genetic diversity across entire gene segments by computing the statistics π N and π S (for details, see Methods). π N , or nonsynonymous diversity, describes the frequency of mutations within a virus population that encode an amino-acid change. Similarly, π S , or synonymous diversity, describes the frequency of silent mutations. Comparing these statistics for a given gene segment provides information about the ‘direction’ of natural selection. Generally, a π N /π S ratio >1 indicates that positive selection is favoring genetic diversification. By contrast, a π N /π S ratio <1 indicates that purifying (or negative) selection is acting to maintain a ‘fit’ consensus sequence by removing deleterious mutations. Performing pairwise comparisons of π N or π S across gene segments (for example, comparing statistics for HA and NA within one virus sample, or for the HAs of two different viruses) provides information about the relative genetic diversity of any pair of gene segments. It is important to reiterate here that our experiment uses a reassortant virus expressing an avian HA but all other viral gene segments from a mammalian-adapted pandemic H1N1 virus; the results of these analyses may therefore differ when applied to fully avian viruses. We compute overall π N and π S in each animal using combined sequence data from every available time point. In HA, overall means of π N and π S do not differ significantly either in index animals or in contact animals when all time points are considered together ( Fig. 5a,b ; compare dark blue and light blue or dark red and light red bars). This result suggests that, although positive selection is likely acting at specific sites, such as nucleotide 788 in index animals, it is not driving diversification throughout the HA gene. In NA and M1, the overall mean π S is often higher than the mean π N in both index and contact animals ( Fig. 5a,b ; compare dark blue and light blue bars or dark red and light red bars). This result indicates that nonsynonymous mutations in NA and M1 are generally removed by purifying selection and therefore remain at low frequencies in the virus population in index animals. Together, these data suggest that different selective pressures act on HA, as compared with NA and M1, during replication and transmission of reassortant H5N1 viruses in ferrets. 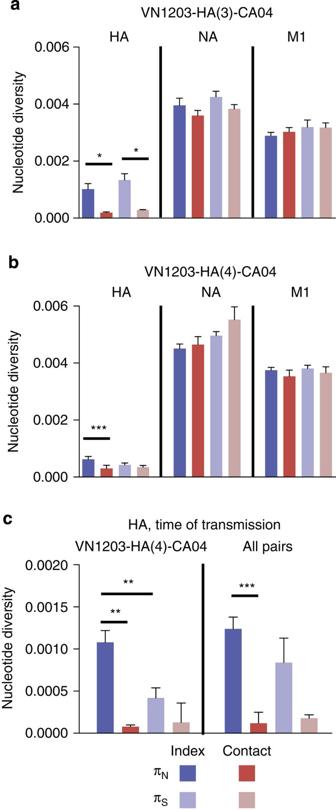Figure 5: Within-host nucleotide diversity in HA. We determine the mean nonsynonymous (πN) and synonymous (πS) nucleotide diversity throughout the experiment in the HA, NA and M1 coding regions of viruses isolated from index and contact ferrets infected with (a) VN1203-HA(3)-CA04;n=2 or (b) VN1203-HA(4)-CA04;n=4. (c) To independently assess the impact of transmission on HA nucleotide diversity, we compared πNand πSat the single time point closest to transmission for each ferret pair. For this analysis, we considered either the VN1203-HA(4)-CA04-infected group alone (c, left) or all six ferret pairs together (c, right). In each graph, vertical bars represent the mean nucleotide diversity for all index and contact samples; error bars represent s.e.m. Dark and light blue bars indicate πNand πS, respectively, in index animals; dark and light red bars indicate πNand πS, respectively, in contact animals. We used pairedt-tests to compare πNand/or πSvalues within and between gene segments. Horizontal bars highlight comparisons for which two values are significantly different. *P<0.05; **P<0.01; ***P<0.001. Figure 5: Within-host nucleotide diversity in HA. We determine the mean nonsynonymous (π N ) and synonymous (π S ) nucleotide diversity throughout the experiment in the HA, NA and M1 coding regions of viruses isolated from index and contact ferrets infected with ( a ) VN1203-HA(3)-CA04; n= 2 or ( b ) VN1203-HA(4)-CA04; n =4. ( c ) To independently assess the impact of transmission on HA nucleotide diversity, we compared π N and π S at the single time point closest to transmission for each ferret pair. For this analysis, we considered either the VN1203-HA(4)-CA04-infected group alone ( c , left) or all six ferret pairs together ( c , right). In each graph, vertical bars represent the mean nucleotide diversity for all index and contact samples; error bars represent s.e.m. Dark and light blue bars indicate π N and π S , respectively, in index animals; dark and light red bars indicate π N and π S , respectively, in contact animals. We used paired t -tests to compare π N and/or π S values within and between gene segments. Horizontal bars highlight comparisons for which two values are significantly different. * P <0.05; ** P <0.01; *** P <0.001. Full size image In our initial analyses, the average values for π N and π S in HA in index ferrets were higher than those in contact ferrets; however, these differences did not attain statistical significance for every pairwise comparison ( Fig. 5a,b ). To more closely examine the impact of transmission on HA genetic diversity, we therefore compare values for π N and π S in HA in index and contact animals, considering only the time points closest to the transmission event. As only two ferret pairs were infected with VN1203-HA(3)-CA04, we cannot perform statistical analyses on that virus alone. We therefore first consider only animals infected with VN1203-HA(4)-CA04 ( Fig. 5c , left side of panel). In this group, the mean π N for the transmitted virus in contact ferrets (0.00008±0.00002) is significantly lower than that found in the virus replicating in index ferrets just before transmission (0.00108±0.00014; P= 0.008, Student’s t -test). Likewise, near the time of VN1203-HA(4)-CA04 transmission, the mean π S is lower in contact than in index animals, although in this case the difference is not statistically significant. Considering all six ferret pairs regardless of infecting virus, the mean π N for the transmitted virus in contact animals (0.00012±0.00013) is significantly lower than the mean π N in the index ferrets near the time of transmission (0.00124±0.00014; P <0.001, Student’s t -test; Fig. 5c , right side of panel, compare dark blue to dark red bars). Similarly, the mean π S value of contact animals is lower than that of index animals near the time of transmission, although this difference narrowly escapes statistical significance ( P= 0.054, Student’s t -test; Fig. 5c , right side, compare light blue to light red bars). Interestingly, when we considered the HA nucleotide diversity in index animals just prior to the estimated time of transmission, the mean of π N for the four index ferrets infected with VN1203-HA(4)-CA04 (0.00108±0.00014) was significantly greater than the mean of π S for the same four animals (0.00042±0.00012; P= 0.004, Student’s t -test; Fig. 5c , left side of panel, compare dark blue to light blue bars), suggesting that HA is undergoing positive selection during the infection of index animals. Together, these results confirm that transmission of these H5N1 viruses to contact animals is associated with a significant reduction in the overall HA nucleotide diversity. We also compute an overall π N and π S for HA, NA and M1 in the stock viruses, finding that π N and π S are in general lower than the values seen in the viruses infecting all the six index animals ( Supplementary Table S8 ). In the case of HA, both π N and π S are significantly lower in stock viruses than in virus from index animals ( P <0.01 in each case, Student’s t -test; Supplementary Table S8 ). In the case of NA and M1, π N and π S are lower in stock viruses than in viruses from the index animals; however, the differences are not statistically significant ( Supplementary Table S8 ). Additionally, π N is lower than π S for the HA, NA and M1 genes of each stock virus, providing the evidence that positive selection on HA sequences did not occur during production of the virus stocks. Together, our data therefore show that there is a dramatic reduction in genetic diversity in HA but not NA or M1, following droplet transmission of H5N1 reassortant viruses, whereas there is no evidence for a similar reduction in diversity following direct inoculation of index animals with stock viruses. Acquisition of a human-transmissible phenotype by H5N1 avian influenza viruses represents a major pandemic threat [2] , [3] , [26] , [27] , [28] . Despite the identification of specific mammal-adapting mutations in the HA genes of H5N1 viruses [2] , [3] , the strength and nature of evolutionary barriers to such adaptation remain unclear [29] . Importantly, few models have measured the impact of within-host ‘quasispecies’ diversity on influenza virus evolution. Here we use deep sequencing to evaluate the impact of viral variation on H5N1 influenza virus host adaptation and mammalian transmission dynamics. Our analyses show that the selection on HA has a main role in driving a bottleneck during the transmission of these reassortant H5N1 influenza viruses among mammals. Together, our results suggest that selection could drive the establishment of infection in mammals by viruses bearing ‘favourable’ HA genes, even when such viruses are in the minority in the source population. Restriction of influenza viral genetic diversity in contact animals likely reflects the various mechanical and immunological barriers to replication that viruses must overcome upon mucosal transmission. This bottleneck could result from the founder effect—that is, a dramatic reduction in effective viral population size without the action of natural selection—and/or from a selective sweep, in which viruses with specific traits are best able to transmit. Influenza virus quasispecies dynamics during transmission has not been well characterized; however, transmission of other diverse RNA viruses has been shown to dramatically reduce quasispecies diversity. In HIV transmission, infection via the cervicovaginal mucosa is initiated by only 1–2 virus clones [30] , [31] , [32] . This bottleneck may be due largely to the founder effect, although HIV variants bearing envelope proteins capable of using CCR5 as a co-receptor for cellular entry appear to be favoured [33] . The transmission of hepatitis C virus is also associated with a genetic bottleneck, which may result from a selective sweep acting on the viral envelope glycoprotein [34] , [35] . By controlling the viral dose administered to naive ferrets via aerosolized droplets, Gustin et al . [36] demonstrated that influenza virus infection can be established by a dose as small as 4 p.f.u., suggesting that the founder effect could reduce viral diversity during influenza transmission by respiratory droplets. Additionally, the anatomic location of replication of variant virus populations in the source host may affect the ‘availability’ of specific virus variants for transmission, providing a further potential mechanism for founder effects to influence the diversity of viruses in individuals infected by respiratory droplets. In our experiment, however, HA diversity was reduced to a much greater extent than diversity in genes encoding NA or M1, suggesting that a selective sweep acted to favour transmission and/or replication of only a subset of HA sequences from index animals in contacts infected by respiratory droplets. Although our results highlight a role for natural selection in determining the composition of HA sequences infecting contact animals, the potential impact of extremely low infecting doses or other factors in the bottleneck associated with transmission cannot be excluded. Although we detect only 1–2 HA ‘haplotypes’ early after infection in contact animals, no single haplotype was consistently associated with transmission ( Fig. 4 ). Perhaps this is because the main determinants of mammalian transmissibility of these reassortant viruses are the mutations identified in our previous study [2] , which were fixed in the virus populations. The haplotypes we identified therefore existed in a background of fixed mutations that already facilitated mammalian transmission of these viruses. Our results suggest that additional amino-acid substitutions may render individual viruses with this genetic background more or less fit for transmission. The specific HA haplotype that establishes infection in naive contact ferrets may vary depending on a number of factors, including the unique constellation of viruses that co-exist in the inoculated ferret because of random mutation and intrahost selective pressures during infection, the titre of each variant virus in the inoculated ferret as the infection progresses, the anatomic location at which each variant virus is replicating and the timing of expulsion of respiratory droplets as it relates to the dynamically changing population of viruses in the inoculated ferret. Further work will therefore be required to understand the nature of selection pressures acting to restrict HA sequence diversity during H5N1 virus transmission among mammals. Replication and transmission of purely avian H5N1 viruses in mammals may result in patterns of selection that differ from those we have observed here using a reassortant virus composed of altered versions of the HA gene segment from an H5N1 virus and seven remaining gene segments from a human H1N1 virus. Notably, adaptive mutations in gene segments other than HA can also affect the ability of purely avian viruses to productively infect mammalian cells [11] , [13] , [37] , [38] . In particular, a lysine residue at PB2 amino acid 627 has consistently been associated with enhanced replication of avian-origin influenza viruses in mammals [3] , [16] , [21] , [22] , [39] , [40] , [41] , [42] . In our study, we observed very little diversification of the NA and M1 genes during the infection of index or contact ferrets ( Supplementary Tables S4 and S6 ) when compared with the H5 HA, perhaps because in our reassortant viruses these gene segments were already well adapted to replicate in mammals. The signatures of purifying selection we observed in these segments (that is, levels of synonymous diversity that were higher than levels of nonsynonymous diversity) are consistent with this interpretation. RNA viruses are characterized by high mutation rates, leading to the accumulation of deleterious mutations, whereas their short replication times and frequently large effective population sizes act to increase the efficacy of purifying selection; that is, as virus titres increase, so does the likelihood that purifying selection will act to remove deleterious mutations from the population [25] , [43] , [44] . Consistent with this model, in HA genes we detected only a small number of sites at which nonsynonymous substitutions accumulated to detectable levels. Positive selection may have acted on these particular sites to enhance viral fitness. For example, we found that low-frequency SNPs encoding alanine-to-serine or alanine-to-threonine substitutions at H5 amino acid 238 (residue 242 by H3 numbering) in the virus stocks rapidly increased in frequency in all the six index animals we examined. Each substitution creates a potential site of N-linked glycosylation within the HA globular head, although the impact of glycosylation at this site (H5 amino acid 236; H3 amino acid 240) has not been characterized. Notably, we found that viruses encoding a serine or threonine at position 238 were not consistently transmitted to contact animals, despite their high frequency in index animals. We speculate that the biological function of serine/threonine 238 may enhance virus replication within mammals but does not favour transmission between hosts. Together, these observations suggest that different viral characteristics, such as transmissibility and replication, may have distinct effects on evolutionary fitness, so that, for example, mutations providing optimal advantages for transmission may exact a cost to replicative capacity. Finally, our findings also suggest that influenza surveillance efforts based on Sanger sequencing may fail to detect the early emergence of genetic markers associated with transmissibility or virulence in mammals, as others have recently speculated [29] . The use of Sanger sequencing for influenza surveillance typically defines consensus sequences, cannot resolve variants present below 20% of the viral population and cannot provide information regarding the genetic linkage of variant nucleotides. As described above, our deep sequencing revealed substantial diversification of HA haplotypes during the infection of index animals. In some instances, the transmitted HA variant was present at frequencies as low as 5.9% in the source animal near the time of transmission, a level below the ability of population-based Sanger sequencing to resolve SNPs [45] . Our results therefore demonstrate that low-level viral variants in the source viral population can nonetheless found infections in new hosts. This finding has important implications for surveillance activities aimed at detecting naturally occurring variants that may have the ability to replicate in and transmit among mammals. Importantly, Sanger sequencing may not only fail to detect biologically relevant viral species in a mixed population but may also define a viral consensus sequence that does not exist in nature. Deploying deep sequencing approaches in surveillance may therefore dramatically enhance our understanding of influenza virus population diversity in reservoir hosts. Infection and transmission in ferrets Studies of H5N1 reassortant virus transmission in ferrets were conducted previously [2] . We summarize the approach for those experiments here to aid the reader in understanding the design of the experiments from which we obtained the samples used for analysis in the present study. Ten-month-old female ferrets ( Mustela putorius furo ) were obtained from Triple F Farms (Sayre, PA, USA). Index ferrets were intranasally inoculated with 10 6 p.f.u. of the indicated virus in 500 μl phosphate-buffered saline. Viruses used were 7:1 reassortant viruses composed of the HA gene segment from A/Vietnam/1203/2004 (VN1203) H5N1, with the indicated mutations and the remaining seven gene segments from A/California/04/2009 (CA04) H1N1 virus. For transmission experiments, ferrets were housed in adjacent transmission cages that prevented direct and indirect contact between animals but allowed spread of influenza virus through the air (Showa Science, Chiyoda-ku, Japan). Twenty-four hours after infection, one naive ‘contact’ ferret was placed in a transmission cage adjacent to the index ferret. Nasal washes were collected from index and contact ferrets on day 1 after inoculation or co-housing, respectively, and then every other day subsequently ( Supplementary Fig. S2 ). Viral loads in nasal washes were determined using the standard plaque assay on MDCK cells using serially diluted nasal wash fluid. Animal studies were performed in accordance with the Animal Care and Use Committee guidelines of the University of Wisconsin—Madison. Biosafety and biosecurity All biosafety protocols, including those for isolation and sequencing of viral nucleic acids, were approved by the University of Wisconsin—Madison’s (UW’s) Institutional Biosafety Committee after risk assessments conducted by the UW Office of Biological Safety. In addition, the UW Biosecurity Task Force regularly reviews the research programme and ongoing activities of the UW Influenza Research Institute (IRI). The task force has a diverse skill set and provides support in the areas of biosafety, facilities, compliance, security and health. Members of the Biosecurity Task Force are in frequent contact with the principal investigator and personnel of the IRI to provide oversight and assure biosecurity. Isolation of RNA from samples containing H5N1 reassortant viruses was performed in enhanced BSL3 containment laboratories approved for such use by the CDC and the USDA following procedures approved by the UW Office of Biological Safety. RNA was isolated using techniques documented to inactivate virus particles in samples before the removal from the BSL3 laboratory space. DNA library preparation and sequencing were performed in a BSL2 laboratory space. Amplification of genomic material for deep sequencing Total RNA was purified from nasal wash fluid using the RNeasy Mini Kit (Qiagen, USA). Viral RNA encoding the HA, NA and M gene segments were reverse transcribed using the Superscript III reverse transcriptase (Invitrogen, USA) according to the manufacturer’s instructions and the primer 5′-AGCAAAAGCAGG-3′. The resultant cDNA was used as template in a PCR reaction to amplify the HA, NA and M gene segments using the following primer pairs (see Supplementary Table S9 for primers) and the high fidelity iProof polymerase and buffers (Bio-Rad, USA). PCR was performed by incubating the reaction mixtures at 94 °C for 2 min, followed by 35 cycles of 94 °C for 30 s, 62 °C for 30 s and 72 °C for 2 min, followed by a final extension step at 72 °C for 10 min. PCR products were separated using electrophoresis on a 1% polyacrylamide gel. The band corresponding to the full-length amplified gene segment was excised and the DNA-recovered using the QIAquick Gel Extraction Kit (Qiagen, USA). Illumina MiSeq Sequencing Amplified gel-purified PCR products were quantified using the Qubit dsDNA High Sensitivity Kit (Invitrogen, USA) and diluted in DEPC-treated water to a final concentration of 2.5 ng μl −1 . Samples were prepared for sequencing on the Illumina MiSeq platform using the Nextera DNA Sample Preparation Kit according to the manufacturer’s instructions with slight modifications. Individual sample preparation reactions were performed for each HA amplicon, whereas the NA and M amplicons generated for each individual animal at each time point were combined and processed together. The prepared DNA was purified with Zymo DNA Clean and Concentrator Spin Columns and eluted in 25 μl resuspension buffer. Dual DNA bar codes (Epicentre, USA) were added to each sample reaction using limited-cycle PCR to enable multiplexed sequencing of prepared DNA samples. Limited-cycle PCR products were purified using a 0.375 × AMPure XP bead cleanup (Beckman Coulter, USA) and eluted in 32.5 μl of the AMPure XP resuspension buffer. Eluted DNA was quantified using the Qubit dsDNA High Sensitivity Kit (Invitrogen, USA), and the average fragment length was determined using the Agilent High Sensitivity Bioanalyzer Kit. Fragmented and indexed samples were pooled in equimolar amounts into two separate 2 nM libraries for sequencing on the Illumina MiSeq. Prepared samples were split into two sequencing runs to ensure an adequate depth of coverage to detect low-frequency viral variants. The sample libraries were denatured into single-stranded DNA by mixing with an equal volume of 0.1 N NaOH for 5 min, and were then diluted to 20 pM using the supplied HT1 buffer (Illumina, USA). Denatured 20 pM libraries were then diluted to 6 pM with 2% phiX control library added to run quality assurances. Six hundred microlitre was loaded into a 300-cycle reagent cartridge. Illumina MiSeq run settings were entered into sample sheets using the Illumina Experiment Manager software v1.3.66 as the following: Workflow: DenovoAssembly; Assay: Nextera; Chemistry: Amplicon; and Reads: 160 × 160 with automatic adapter removal. Sequence information was stored as fastq-formatted data and used for further analysis. Quality trimming and assembly of Illumina MiSeq data Illumina MiSeq sequences were imported into CLC Genomic Workbench, Version 5.1 (CLC bio, Denmark). Sequence reads were deconvoluted using the DNA indices that were introduced during the limited cycle PCR stage of sample preparation as described above. Reads were trimmed using a quality-limit threshold of 0.001 and reads, regardless of mate pair, >100 base pairs in length were retained. Sequence ‘reads’ for each sample were mapped to a full-length HA, NA or M reference sequence. SNP detection SNPs were called using CLC Genomic Workbench, Version 5.1 using all available sequencing data with at least 100 sequence reads covering each nucleotide position and a central base quality score of Q30 or greater. The Geneious bioinformatic software suite, Version 5.6.3 (Biomatters, Ltd., New Zealand) was used as an independent method of calling SNPs to ensure call reproducibility. Geneious variant calling occurred only at sites inside the coding regions with read coverage >100. For each analysis, SNPs occurring in only one sequence read—that is, ‘singleton SNPs’— were discarded. No minimum variant frequency threshold was used and approximate variant P -values were calculated. SNP-detection limit validation The M gene segment of the seasonal H1N1 virus A/Kawasaki/173/2001 was amplified with the help of PCR using Phusion DNA Polymerase (New England Biolabs, UK). The resulting cDNA was cloned using the Zero Blunt Cloning kit (Invirogen, USA). The presence of the K173 M gene insert in plasmid DNA was verified by sequencing. The K173 M gene-containing plasmid was used as template for an in vitro transcription reaction using the MEGAscript T7 Kit (Life technologies, USA). K173 M gene transcripts were purified using phenol/chloroform extraction. To evaluate the error rate of our library preparation and deep sequencing, we used the K173 M gene transcripts and the K173 M gene-containing plasmid as starting templates. The K173 M gene transcript was reverse-transcribed using the Superscript III reverse transcriptase (Invitrogen, USA) according to the manufacturer’s instructions and the primer 5-AGCAAAAGCAGG-3′. The resultant K173 M gene cDNA and the plasmid-encoded K173 M gene were used as input template (100,000 copies of each template total) to amplify a 430 base pair product using the high-fidelity iProof polymerase and buffers (Bio-Rad, USA) with the following primer pairs (see Supplementary Table S9 for primers). PCR was performed with an initial step at 94 °C for 2 min, followed by 35 cycles of 94 °C for 30 s, 62 °C for 30 s and 72 °C for 2 min, followed by a final extension step at 72 °C for 10 min. The amplicon was gel-purified using the QIAquick Gel Extraction Kit (Qiagen, USA). Extracted DNA was prepared for sequencing using the Nextera XT DNA Sample Preparation Kit and sequenced on the Illumina MiSeq as described above. Quality trimming, assembly and SNP detection of Illumina MiSeq data were performed as described above. SNP and mapping statistics were calculated using R version 2.15.1 ( http://www.R-project.org/ ). Enumeration of Linked SNPs within HA gene segments The PERL programming language was used to design a novel method of mining paired-end sequence data for linked nucleotide polymorphisms. Our script LinkGE was used to enumerate linked polymorphisms within a predefined query set. Query nucleotide positions used for LinkGE were included if they met the following three criteria: (a) SNPs fell within a defined window of ~500 base pairs to accommodate analysis of paired end reads within the physical constraints of library fragment distribution and average sequence read length; (b) SNPs were not fixed—that is, <100% of sequence reads were identical to each other; (c) SNPs were detected at or above 1% of all reads at any time point in any animal. Parameter files were independently generated for both transmission groups. CLC Genomic Workbench-generated assemblies were used as input data for the LinkGE script, and the frequencies of each constellation of linked polymorphisms were determined. Constellations of linked polymorphisms, which we call ‘haplotypes’, produced using LinkGE were manually confirmed within the original assemblies. To further validate the identity of haplotypes and their frequencies within the bulk viral population as determined using LinkGE, the HA gene segments from samples collected at a single time point of two pairs of ferrets used in the transmission experiment were independently reverse-transcribed, PCR-amplified and cloned using the Perfectly Blunt Kit (EMD Millipore, USA). The HA gene segments contained within individual plasmids were sequenced using a conventional Sanger chain-termination sequencing approach and compared with the results produced through the analysis of paired-end deep sequencing data using LinkGE. The LinkGE source code is freely available on http://dholk.primate.wisc.edu/project/dho/public/LinkGe/begin.view . Calculation of nucleotide diversity estimates To measure nucleotide sequence diversity in HA, NA and M1 genes, we first used deep sequencing ‘reads’ from each animal to estimate the number of synonymous substitutions per synonymous site ( d S ) and the number of nonsynonymous substitutions per nonsynonymous site ( d N ). The numbers of synonymous and nonsynonymous sites in each coding sequence were estimated following the method of Nei and Gojobori [46] . Sequence heterogeneity across entire gene segments was then estimated by computing synonymous nucleotide diversity (π S ), defined as the mean of d S for all pairwise comparisons among a set of sequences, and nonsynonymous nucleotide diversity (π N ), which is the mean of d N for all pairwise comparisons among a set of sequences. Note that this method compares sequence ‘reads’ from an individual sample to each other and does not use a consensus or other external references as a basis for comparison. As most random amino-acid-changing mutations are likely to be disadvantageous, we expect that π N will equal π S under strict neutrality. If π N exceeds π S for a gene segment, this indicates that selection is acting to favour nonsynonymous mutations. We therefore used paired t -tests to evaluate the hypothesis that π N =π S within genes, or that, for example, π N of one gene equals π N of another. How to cite this article: Wilker, P. R. et al . Selection on haemagglutinin imposes a bottleneck during mammalian transmission of reassortant H5N1 influenza viruses. Nat. Commun. 4:2636 doi: 10.1038/ncomms3636 (2013).